Plasmonic black gold by adiabatic nanofocusing and absorption of light in ultra-sharp convex grooves Excitation of localized and delocalized surface plasmon resonances can be used for turning excellent reflectors of visible light, such as gold and silver, into efficient absorbers, whose wavelength, polarization or angular bandwidths are however necessarily limited owing to the resonant nature of surface plasmon excitations involved. Nonresonant absorption has so far been achieved by using combined nano- and micro-structural surface modifications and with composite materials involving metal nanoparticles embedded in dielectric layers. Here we realize nonresonant light absorption in a well-defined geometry by using ultra-sharp convex metal grooves via adiabatic nanofocusing of gap surface plasmon modes excited by scattering off subwavelength-sized wedges. We demonstrate experimentally that two-dimensional arrays of sharp convex grooves in gold ensure efficient (>87%) broadband (450–850 nm) absorption of unpolarized light, reaching an average level of 96%. Efficient absorption of visible light by nanostructured metal surfaces open new exciting perspectives within plasmonics, especially for thermophotovoltaics. Early blackened metallic surfaces produced by the distillation of metals at relatively high pressures [1] , as well as recent blackening of metals [2] , [3] and silicon [4] caused by intense laser irradiation, suppress reflection of light through a combined effect of nano-, micro- and macro-structured surface morphology, resulting in strong multiple light scattering and absorption. Even though laser-induced blackening of materials results in very efficient and broadband light absorption, characterization and reproduction of the resulting surface topography down to all fine details is essentially impossible, rendering quantitative descriptions of this effect beyond using statistical averages very difficult. Metal nanostructures supporting surface plasmon (SP) modes constitute a new class of promising candidates for designing efficient absorbers with well-defined geometries [5] , [6] . For this purpose, one can exploit excitation of localized and delocalized SP resonances, thereby facilitating coupling of incident light to strongly confined SP modes that are absorbed by the metal. Efficient resonant light absorption by various plasmonic structures, including microcavities [7] , lamellar gratings [8] , [9] and gap SP resonators [10] , [11] , [12] , has been demonstrated, exhibiting, however, inevitable wavelength, angle or polarization sensitivity due to the resonant nature of SP excitations. Nonresonant (broadband) absorption of linearly polarized and unpolarized light has been demonstrated with plasmonic composite metamaterials involving a nanostructured metallic layer shaped in the form of a deep diffraction grating [13] and metal nanoparticles embedded in dielectric layers [14] , [15] , respectively. As far as individual nanostructures are concerned, nonresonant absorption by touching subwavelength-sized metal cylinders [16] and spheres [17] , as well as with optical analogues of black holes based on metamaterials [18] , [19] and gap SP modes [20] , has been proposed and theoretically analysed. Apart from fundamental challenges in turning shiny metals black, suppression of light reflection is of great current interest for both photovoltaics [6] and thermophotovoltaics [21] . In the latter case, one would prefer to achieve efficient broadband absorption and, according to Kirchhoff's law, emission of visible light with homogeneous materials so as to avoid thermal stresses due to different thermal expansion properties. Nonresonant absorption by touching subwavelength-sized metal cylinders [16] and spheres [17] is broadband but relatively inefficient for wavelengths longer than the SP resonance wavelength, with the absorption cross-section becoming much smaller than the geometrical one [16] , [17] . At the same time, complete absorption of gap SP modes has been shown to be possible near the contact area of macroscopic spherical surfaces [20] . Here we realize nonresonant light absorption with nanostructured metal surfaces by making practical use of one of the most intriguing and fundamental phenomena in plasmonics—nanofocusing of optical energy in tapered plasmonic waveguides [22] , [23] . We demonstrate that one- and two-dimensional (1D and 2D) arrays of ultra-sharp convex metal grooves lead to efficient broadband light absorption via adiabatic nanofocusing of gap SP (GSP) modes excited by scattering off subwavelength-sized wedges. Theoretical background Let us consider a 1D array of grooves in metal illuminated with a monochromatic plane wave ( Fig. 1a ). For subwavelength array periods and p -polarized incident light (in which the electric field is perpendicular to the groove direction for the discussed geometry), excitation of GSP modes propagating inside the grooves (towards the bottom) is expected. Complete absorption of these modes is possible, if the regime of adiabatic nanofocusing is realized throughout the groove, that is, if variations of the GSP propagation constant inside a tapered groove are small on the scale of the light wavelength [23] , [24] . The adiabatic GSP nanofocusing results thereby in the GSP propagation without reflection towards the groove bottom, where GSP modes asymptotically stop, dissipating eventually in the metal [24] . This (nonresonant and broadband) scenario is similar to those of radiation nanofocusing by tapered nanowires [23] and touching spherical surfaces [20] . It has however been shown that the GSP nanofocusing in linearly tapered gaps, that is, in (individual) V-grooves, is resonant and does involve GSP reflections by groove walls [25] . Consequently, light reflection by periodic 1D [26] and 2D [27] V-groove arrays was found to be resonant as well, being sufficiently low only within limited wavelength ranges. Let us explore in more detail the condition for adiabatic nanofocusing [23] , [24] by making use of the (approximate) explicit relation for the GSP propagation constant [28] , which is well established [25] . It can be shown (similar to what has been done for touching spherical surfaces [20] ) that the adiabatic condition can be cast in the following form (for details, see Methods): where q is the real part of the GSP propagation constant, λ is the light wavelength in air, w ( z ) is the groove width at the depth coordinate z ( Fig. 1b ), ɛ d and ɛ m =− ɛ′ + iɛ ″ are the dielectric constants of the dielectric and the metal, respectively. The obtained relation implies that, in the case of V-grooves (that is, when d w /d z =constant), the adiabatic condition would inevitably break down near the groove bottom, where the groove width becomes sufficiently small, causing GSP reflection and resonant response [25] , [26] , [27] . The condition can still be satisfied throughout the whole groove depth for the configuration of convex metal grooves with the groove walls becoming parallel at the contact point, for example, being formed by touching segments of cylinders. In the case of cylinders with equal radii R , the adiabatic condition reduces to which is, in practice, met for radii much larger than the light wavelength ( Supplementary Fig. S1 ). 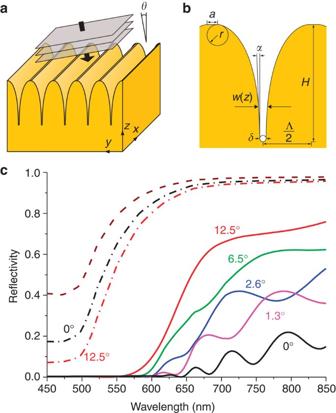Figure 1: Reflection of light by 1D groove arrays. (a) Schematic of the considered configuration, showing orientation of a groove array and incident plane wave, whose phase fronts are represented by grey squares on the arrow indicating the propagation direction of incident light. (b) Geometrical parameters defining the profile of groove arrays. (c) Reflectivity spectra calculated for 250-nm-period arrays of 500-nm-deep grooves with the following parameters kept constant:a=r=10 nm. Solid lines correspond to the reflection spectra ofp-polarized light (which in our case is polarized along theyaxis) calculated for normal incidence (θ=0°) and a minimum gap widthδ=0.3 nm (which is close to the gold atom diameter), and for different inclination angles:α=0, 1.3, 2.6, 6.5 and 12.5°. Reflectivity spectrum for a flat gold surface is shown with a dashed line. Reflectivity spectra fors-polarized (which, in our case, is polarized along thexaxis at normal incidence) light are shown with dash-dotted lines for two limiting inclination angles:α=0 and 12.5°. Gold dielectric constants are taken from Johnson and Christy29. Figure 1: Reflection of light by 1D groove arrays. ( a ) Schematic of the considered configuration, showing orientation of a groove array and incident plane wave, whose phase fronts are represented by grey squares on the arrow indicating the propagation direction of incident light. ( b ) Geometrical parameters defining the profile of groove arrays. ( c ) Reflectivity spectra calculated for 250-nm-period arrays of 500-nm-deep grooves with the following parameters kept constant: a = r =10 nm. Solid lines correspond to the reflection spectra of p -polarized light (which in our case is polarized along the y axis) calculated for normal incidence ( θ =0°) and a minimum gap width δ =0.3 nm (which is close to the gold atom diameter), and for different inclination angles: α =0, 1.3, 2.6, 6.5 and 12.5°. Reflectivity spectrum for a flat gold surface is shown with a dashed line. Reflectivity spectra for s -polarized (which, in our case, is polarized along the x axis at normal incidence) light are shown with dash-dotted lines for two limiting inclination angles: α =0 and 12.5°. Gold dielectric constants are taken from Johnson and Christy [29] . Full size image These guidelines for achieving nonresonant radiation absorption by adiabatic GSP nanofocusing thus require subwavelength-period arrays of convex grooves in metals that are infinitely sharp at the bottom, so that both the groove width w ( z ) and the wall inclination angle approach zero towards the groove bottom. Although the latter requirement is crucial for cancelling completely the GSP reflection, it is clearly not possible to achieve in practice. In our 2D simulations based on the Green's function surface-integral equation method [26] , we have used cylindrical segments to represent the groove walls approaching each other down to a minimum gap of width δ at the groove bottom (rounded accordingly) and introduced the wall inclination angle α so that d w /d z 2 α at the rounding point ( Fig. 1b ). We have found, that for realistic wedges with 10-nm-wide flat tops smoothly connected (with curvature radii of 10 nm) to cylindrical segments, the reflectivity of visible and near-infrared p -polarized light at normal incidence can be suppressed to arbitrarily low levels once the inclination angle α and the minimum gap width δ are sufficiently small ( Fig. 1c ). For non-zero values of these parameters, the reflection spectra exhibit resonant oscillations associated with GSP reflection resulting in interference of counter-propagating GSPs ( Supplementary Fig. S2 ) similar to that observed for V-grooves [25] , [26] . It should be noted that these oscillations are pronounced only for relatively long wavelengths (>550 nm), because, even though SP modes (and thereby GSPs) propagating along gold-air interfaces do exist for shorter wavelengths (but longer than 400 nm), the SP propagation length decreases drastically to submicron distances for short wavelengths (<550 nm) [30] , effectively eliminating the GSP reflection at the groove bottom [25] . Whereas both inclination angle and minimum gap width should be made as small as possible, the minimum gap width is probably the most critical one from the fabrication point of view. We have however found that, whereas the array reflectivity at long wavelengths increases rapidly when increasing the minimum gap width, this increase can be somewhat compensated by using deeper grooves ( Supplementary Fig. S3 ). As far as the influence of the angle θ of incidence is concerned, the main effect for relatively small angles ( θ <40°) and subwavelength array periods ( Λ ≤ λ /2) is in blue-shifting the wavelength-dependent reflectivity oscillations ( Supplementary Fig. S4 ). For larger angles of incidence, the reflectivity levels become progressively larger in the whole wavelength range, as the GSP excitation efficiency decreases rapidly when the incident field phase variation Δφ across one period, Δφ =(2 π / λ )· Λ sin θ , becomes significant. To conclude the theoretical considerations, it should be noted that sub-nanometre-sized gap widths might not even be practical to realize, and that nanometre-sized gap widths already call for a description beyond the common local-response approximation [30] . On the other hand, various nonlocal effects, which are detrimental for reaching giant field enhancements in tiny gaps and at sharp edges, can be, in our case, rather useful as these effects would generally increase the light absorption [31] . A recent analysis (conducted in the near-field approximation) of nonlocal effects in the configuration of touching nanowires [32] indicated that spatial dispersion opens a possibility for plasmonic modes to sneak past the touching point as well as to excite longitudinal plasmons. In our configuration, these effects imply that the reflectivity spectra for vanishingly small gap widths δ would still feature resonant oscillations somewhat similar to those obtained for non-zero gap widths δ , but with significantly damped oscillation amplitudes. Finally, it should be mentioned that the 2D simulations described have been compared with 3D simulations conducted using the finite-difference time-domain method for a few sets of configuration parameters, when considering the Gaussian beam illumination, and found in good quantitative agreement. At the same time, modelling of 2D arrays of ultra-sharp grooves turned out to be a very challenging task and currently beyond our capabilities. It is however expected that 2D arrays of touching domes would also ensure adiabatic nanofocusing of GSP modes in a manner similar to that described for touching spherical surfaces [20] . 1D groove arrays For experimental observation of nonresonant radiation absorption by adiabatic GSP nanofocusing, we have fabricated 1D groove arrays (size 35×35 μm 2 ) using focussed ion-beam (FIB) milling of 900-nm-thick gold films deposited on fused silica substrates ( Fig. 2a ). Using single-line milling (with 2 passes), we have successfully fabricated 250- and 350-nm-period arrays of ultra-sharp convex grooves featuring practically parallel walls at the bottom ( Fig. 2b ). Reflectivity spectra measured in the wavelength range of 450–850 nm, with different polarizations of the incident light, have immediately revealed the effect of 'black gold' for p -polarization ( Fig. 2c,d ). The experimental reflectivity spectra shown hereafter were calibrated using a broadband reference mirror so that the reflectivity data are displayed in absolute (not arbitrary) units. The black gold effect was found to be especially pronounced for the 250-nm-period array featuring a ten-fold reduction in the reflectivity (as compared with a flat gold surface) within the wavelength range of 450–730 nm. We have also experimentally observed the effect of non-zero wall-inclination angles α by using 7-line FIB milling for each groove (with 3 passes), in one case (α=14°) with a slightly defocussed ion-beam, to fabricate grooves with profiles closer to that of V-grooves. The corresponding reflectivity spectra were found to be markedly different with the reflectivity rapidly increasing for the wavelengths larger than 550 nm ( Fig. 2d ). In general, the trends observed in the experimental reflectivity spectra are essentially the same as those obtained in simulations apart from relatively large reflectivity levels measured at short (<550 nm) wavelengths ( Figs 1c and 2d ) that can most probably be related to the progressively stronger scattering contribution (scaling as λ −4 ) originating from surface roughness ( Fig. 2a ) that decreases the GSP excitation efficiency. Using the developed technique of fabricating ultra-sharp grooves, we have also studied the influence of the groove depth on the reflection spectra for two different array periods. Gradual blackening of the nanostructured gold areas that also included colour transformations ( Supplementary Fig. S5 ) was observed thus experimentally confirming that the light absorption in subwavelength-period groove arrays occurs independently of the period ( Supplementary Fig. S6 ), that is, absorption takes place separately inside individual grooves as was implicitly assumed in the above qualitative consideration of this effect. It is also worth noting that, due to the relatively small sizes of the fabricated groove arrays, we had to focus the incident radiation with an objective (typically with a numerical aperture (N.A. )=0.9) introducing thereby an angular spectrum of incident directions. We did, however, check that the influence of the numerical aperture used was insignificant ( Supplementary Fig. S6d ). 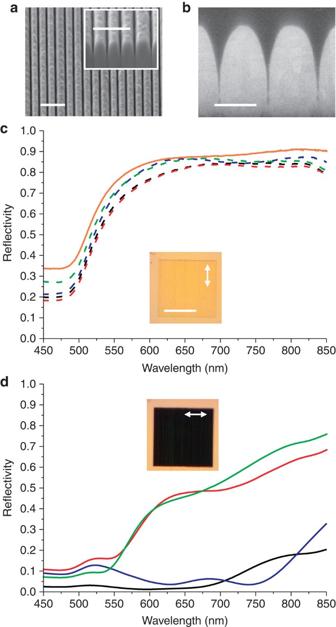Figure 2: Reflectivity of 1D groove arrays in gold. Scanning electron microscopy images of (a) 350-nm-period array of ultra-sharp 450-nm-deep grooves milled in gold (scale bar, 1 μm) displaying slight period variations and surface roughness (see inset), and (b) its cross-section, revealing a convex shape of the grooves (scale bar, 300 nm) and demonstrating negligibly small wall inclination angles,α0° (Fig. 1b). (c,d) Reflectivity spectra of (c)s-polarized (along thexaxis) and (d)p-polarized (along theyaxis) light for 450-nm-deep convex grooves with different inclination anglesαarranged in 1D arrays with different periodsΛ, shown with green (α=14°,Λ=350 nm), red (α=9°,Λ=350 nm), blue (α=0°,Λ=350 nm) and black (α=0°,Λ=250 nm) dashed (s-polarization) and solid (p-polarization) lines. Reflectivity spectrum for a flat gold surface is shown with a solid yellow line inc. Insets display optical microscope images (scale bar, 20 μm) of the 250-nm-period array of ultra-sharp (α0°) 450-nm-deep grooves obtained for two orthogonal polarizations of incident light (polarization directions are indicated with arrows in the insets). Figure 2: Reflectivity of 1D groove arrays in gold. Scanning electron microscopy images of ( a ) 350-nm-period array of ultra-sharp 450-nm-deep grooves milled in gold (scale bar, 1 μm) displaying slight period variations and surface roughness (see inset), and ( b ) its cross-section, revealing a convex shape of the grooves (scale bar, 300 nm) and demonstrating negligibly small wall inclination angles, α 0° ( Fig. 1b ). ( c , d ) Reflectivity spectra of ( c ) s -polarized (along the x axis) and ( d ) p -polarized (along the y axis) light for 450-nm-deep convex grooves with different inclination angles α arranged in 1D arrays with different periods Λ , shown with green ( α =14°, Λ =350 nm), red ( α =9°, Λ =350 nm), blue ( α =0°, Λ =350 nm) and black ( α =0°, Λ =250 nm) dashed ( s -polarization) and solid ( p -polarization) lines. Reflectivity spectrum for a flat gold surface is shown with a solid yellow line in c . Insets display optical microscope images (scale bar, 20 μm) of the 250-nm-period array of ultra-sharp ( α 0°) 450-nm-deep grooves obtained for two orthogonal polarizations of incident light (polarization directions are indicated with arrows in the insets). Full size image 2D groove arrays The successful demonstration of the black gold effect with 1D groove arrays encouraged us to try removing the remaining selectivity in the absorption of light, namely, the polarization selectivity. It turned out, however, that the natural extension of the above experiments by milling 2D arrays of crossed grooves is not that easy to implement because of re-deposition of milled away gold into the already fabricated grooves. The latter was found to result in strong asymmetry of the reflection properties with respect to the polarization direction of the incident radiation ( Supplementary Fig. S7 ). After trying several approaches to circumvent this problem, we have succeeded in fabricating 250- and 350-nm-period 2D arrays with relatively low structural and, thereby, reflection anisotropy ( Fig. 3 ) by milling orthogonally oriented grooves in several passes, while changing the milling direction several times (first two passes along the x -, then two passes along y , and finally one pass along x axis). The FIB milling was terminated once the top level of arrays started to decrease below the flat gold surface level, limiting thereby the groove depths to the values that were smaller than those reached with 1D groove arrays. The colour of the resulting nanostructured gold surfaces was found not to be really black but dark red for the 250-nm-period array ( Fig. 3b,c ) and dark green for the 350-nm-period array, reflecting the occurrence of broad reflection maxima in the corresponding spectra ( Fig. 3d ), which can be associated with localized SP resonances [33] in prolate gold tips ( Fig. 3a ) that enhance light scattering in wave components propagating in free space (away from the sample surface). Nevertheless, the suppression of gold reflectivity below 13% achieved with both arrays as a result of surface nanostructuring for both polarizations in the whole investigated wavelength range of 450–850 nm is a remarkable result, demonstrating the robustness of our approach. In fact, considering only the 350-nm-period arrays of 400-nm-deep grooves brings the average (for both polarizations and within the whole wavelength range of 450–850 nm) reflectivity level down to 4.0%, with the reflectivity variations between 1.9 and 8.6%. Consequently, in the absence of transmission, this reflectivity signifies an average absorption of 96% of unpolarized light in this wavelength range. Finally, we note that the investigated black gold effect has a long-wavelength limit, which is related to both the adiabatic condition (equation (1)) and a general decrease in the plasmon (including GSP modes) absorption for longer wavelengths. This long-wavelength limit of efficient light absorption can however be influenced by adjusting the wall inclination angle ( Figs 1c and 2c ) and the groove depth ( Supplementary Fig. S3 and S6 ). 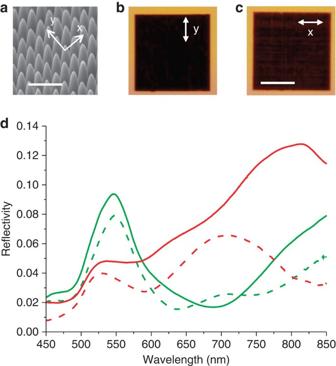Figure 3: Reflectivity of 2D groove arrays in gold. (a) Scanning electron microscopy image (under angled view) of a 250-nm-period array of orthogonally crossed ultra-sharp convex 250-nm-deep grooves milled in gold (scale bar, 700 nm). (b,c) Optical microscope images of the 250-nm-period groove array obtained for two orthogonal polarizations of incident light (scale bar, 7 μm) that are indicated with respect to the axes marked in (a). (d) Reflectivity spectra ofx- (solid lines) andy-polarized (dashed lines) light (as marked ina) for crossed convex grooves of different depthsHarranged in 2D arrays with different periodsΛare shown with green (H=400 nm,Λ=350 nm) and red (H=250 nm,Λ=250 nm) lines. Figure 3: Reflectivity of 2D groove arrays in gold. ( a ) Scanning electron microscopy image (under angled view) of a 250-nm-period array of orthogonally crossed ultra-sharp convex 250-nm-deep grooves milled in gold (scale bar, 700 nm). ( b , c ) Optical microscope images of the 250-nm-period groove array obtained for two orthogonal polarizations of incident light (scale bar, 7 μm) that are indicated with respect to the axes marked in ( a ). ( d ) Reflectivity spectra of x - (solid lines) and y -polarized (dashed lines) light (as marked in a ) for crossed convex grooves of different depths H arranged in 2D arrays with different periods Λ are shown with green ( H =400 nm, Λ =350 nm) and red ( H =250 nm, Λ =250 nm) lines. Full size image We have suggested a new approach for achieving efficient broadband (nonresonant) light absorption with well-defined (homogeneous) metal nanostructures that makes practical use of the phenomenon of nanofocusing of optical energy in tapered plasmonic waveguides [22] , [23] , that is, via adiabatic nanofocusing of GSP modes excited by scattering off subwavelength-sized wedges. Qualitative considerations indicated that complete absorption of light requires the use of subwavelength-period arrays of ultra-sharp convex grooves so as to realize the adiabatic regime of GSP nanofocusing in a manner similar to that described recently for plasmonic black holes [20] . Theoretical analysis of light reflection by 1D groove arrays (conducted using the Green's function surface-integral equation method [26] ) elucidated the influence of different structural parameters on the array absorption efficiency, substantiating the qualitative arguments and highlighting the need for going beyond the local-response approximation in SP modelling. We have fabricated 1D and 2D arrays of ultra-sharp convex grooves in gold and demonstrated efficient broadband (450 – 850 nm) light absorption, reaching an extraordinary low average reflectivity of 4.0%. It should be emphasized that our approach can naturally be exploited with other metals, for example, with nickel that, apart from being much cheaper than gold and having a much higher melting temperature, features stronger plasmon absorption, promising significantly lower reflectivity levels to be achieved with considerably less sharp grooves ( Fig. 4 ) that can be fabricated with more practical techniques, such as nanoimprint lithography and reactive-ion etching [34] . Efficient broadband absorption of radiation in the visible and near infrared by thin nanostructured metal films that can also be strongly polarization selective (with 1D groove arrays) open new exciting perspectives within plasmonics, especially for thermophotovoltaics [12] , [21] . 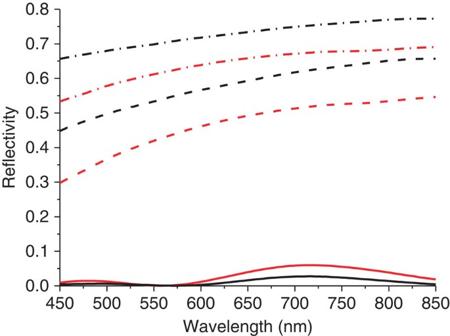Figure 4: Reflectivity of 1D groove arrays. Reflectivity spectra of thes-polarized (along thexaxis) andp-polarized (along theyaxis) light for groove arrays in palladium and nickel and the groove geometry (Fig. 1a) with the parametersa=r=δ=10 nm,H=500 nm,Λ=250 nm, andα=θ=0° are shown with red (nickel) and black (palladium) dashed (s-polarization) and solid (p-polarization) lines, demonstrating that low (<10%) reflectivity levels can be achieved with the grooves fabricated in metals with larger SP losses using relatively low-resolution (~10 nm) techniques. Reflectivity spectra for flat nickel and palladium surfaces are shown with dash-dotted lines. Figure 4: Reflectivity of 1D groove arrays. Reflectivity spectra of the s -polarized (along the x axis) and p -polarized (along the y axis) light for groove arrays in palladium and nickel and the groove geometry ( Fig. 1a ) with the parameters a = r =δ=10 nm, H =500 nm, Λ =250 nm, and α =θ=0° are shown with red (nickel) and black (palladium) dashed ( s -polarization) and solid ( p -polarization) lines, demonstrating that low (<10%) reflectivity levels can be achieved with the grooves fabricated in metals with larger SP losses using relatively low-resolution (~10 nm) techniques. Reflectivity spectra for flat nickel and palladium surfaces are shown with dash-dotted lines. Full size image Adiabatic condition In the following, we show that the adiabatic condition can be expressed in the explicit form as presented in equation (1). We start with considering the (approximate) explicit relation for the GSP propagation constant [28] , which is well established [25] : where q c is the (complex) GSP propagation constant, w is the gap width ( Supplementary Fig. S1a ), k 0 =2 π/λ , with λ being the light wavelength in air, ɛ d and ɛ m =− ɛ ′+ iɛ ″ are the dielectric constants of dielectric and metal, respectively. Considering the GSP propagation in a groove towards its bottom so that the gap (groove) width w ( z ) is decreasing to zero ( Supplementary Fig. S1a ), it is seen that both real and imaginary parts of the GSP propagation constant increase indefinitely, signifying that the GSP asymptotically slows down getting absorbed by the metal. The GSP propagation is adiabatic, that is, occurring without reflection by groove walls, if the GSP propagation constant varies slowly over the light wavelength [23] , [24] : where q is the real part of the GSP propagation constant, that can be written down for 'good' metals, that is, when ɛ ′ ≫ ɛ ″ and ɛ ′ ≫ ɛ d , as follows [equation (2)]: Using equation (4) for the adiabatic condition expressed by equation (3) results (in the limit of w ( z ) → 0, where the GSP propagation constant variations become very strong) in the final representation of the adiabatic condition given by equation (1). Fabrication Arrays of ultra-sharp grooves in gold were fabricated using a cross-beam system (FIB and scanning electron microscope), where a constant current (20–50 pA) of Ga + ions is focussed onto the gold surface at normal incidence, with the position of the beam controlled by a lithography system. To fabricate deep and narrow grooves several consecutive runs (using single-line writing) of each groove are performed. The samples are prepared by depositing 900-nm-thick gold films on a plasma cleaned fused silica substrate by DC sputtering at a deposition rate of 1 Å s −1 . The platinum, which is, in some cases, used to cover the grooves before SEM investigation in the cross-section, is deposited in situ by utilizing a gas injection system and e-beam deposition with the electron column. Optical measurements Reflection properties of the fabricated grooves were studied using spatially resolved linear reflection spectroscopy. The spectroscopic set-up included a BX51 microscope (Olympus) equipped with a halogen light source, polarizers and a fibre-coupled grating spectrometer QE65000 (Ocean Optics). The reflected light was collected in the backscattering configuration using an MPlanFL (Olympus) objective with magnification ×100 (numerical aperture (N.A.)=0.9). The image area analysed by the spectrometer was limited by a pinhole with a diameter of 800 μm resulting in a circular probing area with a diameter of 8 μm. Reflectivity spectra were obtained by using calibration reflection measurements (conducted under the same conditions as those of nanostructured gold surfaces) with a reference broadband laser mirror (Edmund Optics, NT64-114) that exhibits an average reflection of 99% between 350 and 1,100 nm of light wavelength. The microscope images (1,600×1,200 pixels) were captured with a LC20 digital colour camera (Olympus). How to cite this article: Søndergaard, T. et al . Plasmonic black gold by adiabatic nanofocusing and absorption of light in ultra-sharp convex grooves. Nat. Commun. 3:969 doi: 10.1038/ncomms1976 (2012).